Robust absolute magnetometry with organic thin-film devices Magnetic field sensors based on organic thin-film materials have attracted considerable interest in recent years as they can be manufactured at very low cost and on flexible substrates. However, the technological relevance of such magnetoresistive sensors is limited owing to their narrow magnetic field ranges ( ∼ 30 mT) and the continuous calibration required to compensate temperature fluctuations and material degradation. Conversely, magnetic resonance (MR)-based sensors, which utilize fundamental physical relationships for extremely precise measurements of fields, are usually large and expensive. Here we demonstrate an organic magnetic resonance-based magnetometer, employing spin-dependent electronic transitions in an organic diode, which combines the low-cost thin-film fabrication and integration properties of organic electronics with the precision of a MR-based sensor. We show that the device never requires calibration, operates over large temperature and magnetic field ranges, is robust against materials degradation and allows for absolute sensitivities of <50 nT Hz −1/2 . Measuring absolute magnetic fields is crucial for many scientific and technological applications [1] , [2] , [3] ranging from physics to biology. While superconducting quantum interference devices (SQUIDs) address this issue for extremely weak magnetic fields [4] , magnetic resonance (MR)-based sensors allow the drift and offset-free determination of magnetic fields for intermediate to strong magnetic fields. MR magnetometers (MRMs) are based on bringing electromagnetic radiation into MR with paramagnetic centres whose Landé factors are well known [5] , and they exploit Planck's fundamental relationship between the frequency ν of the radiation and the Zeeman energy hν = hγB 0 of the paramagnetic centres to determine a magnetic field ( γ being the gyromagnetic ratio, B 0 the applied magnetic field and h the Planck constant). The drawback of MRMs is their cost and bulkiness: conventional radiation-detected MR requires large volumes (up to hundreds of cubic centimetres) [5] , [6] and as MR signals disappear at low magnetic fields (owing to the disappearance of spin polarization), MRMs are usually poor detectors even for intermediate magnetic field strengths. There have been several proposals to solve these drawbacks by using spin-dependent charge transport or recombination processes in semiconductors for the electrical (EDMR) or optical (ODMR) detection of MR [7] , [8] , [9] . EDMR and ODMR signals usually do not depend on spin polarization [10] , which makes them remarkably sensitive even at very low magnetic fields. In addition, they are not volume sensitive and so can be fabricated on nanoscopic size scales [11] . Previously proposed EDMR- and ODMR-based magnetometers utilized either silicon, whose spin-dependent signals are either entirely absent at room temperature [7] or otherwise very weak, or nitrogen-vacancy centres in diamond, whose optical detection requires a fluorescence microscopy setup [12] , [13] , [14] . In this article, we report on an MRM concept illustrated in Fig. 1, which combines the advantages of organic thin-film electronic devices and traditional MRMs. Specifically, we have investigated the spin-dependent decay of pairs of polarons into excitons in organic diodes based on the π-conjugated organic semiconductor poly(2-methoxy-5-(2′-ethylhexyloxy)- p -phenylene vinylene) (MEH-PPV) [15] , [16] , [17] , [18] ( Fig. 1a ). As this spin-dependent electronic transition governs the material conductivity, MR with either electrons or holes can be detected simply by measuring the current. At its core, the diode as illustrated in Fig. 1a consists of a thin MEH-PPV layer sandwiched between an electron and a hole injecting contact. This structure is identical to those used for conventional organic light-emitting diodes [16] . We have explored the properties of this organic thin-film MRM with regard to its feasibility, its sensitivity and magnetic field limitation as well as its response to temperature fluctuations and device degradation. In the following, the results of these studies are discussed. Unless otherwise stated, the experimental data were acquired at room temperature. 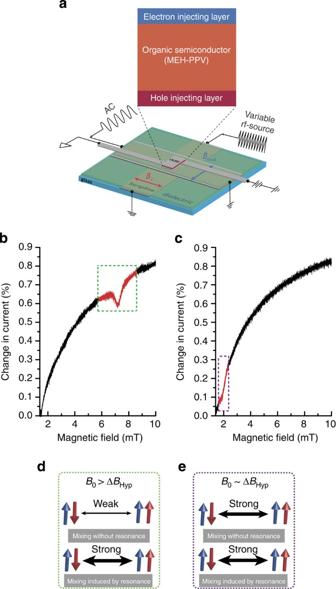Figure 1: Device concept of an organic semiconductor MR-based magnetometer (MRM). (a) The device consists of an organic diode structure (inset, the layers are not to scale), which is located above two mutually perpendicular striplines required for on-chip spin resonant excitation and field modulation. Electron and hole polarons are injected from opposite sides into the diode structure and recombine spin dependently in the organic semiconductor. (b,c) The magnetic field response of a DC current (no modulation) in a bipolar MEH-PPV diode as a function of magnetic field as RF radiation (200 MHz in (b); 50 MHz in (c) is applied. Reductions in the current are seen when MR conditions are satisfied. These are more pronounced when the applied fieldB0>ΔBHypwhere MR-induced spin mixing dominates. (d,e) Schematic illustration of the origin of resistance changes owing to spin mixing induced by the local hyperfine fields (ΔBHyp) and owing to MR excitation. All measurements were performed at room temperature. Figure 1: Device concept of an organic semiconductor MR-based magnetometer (MRM). ( a ) The device consists of an organic diode structure (inset, the layers are not to scale), which is located above two mutually perpendicular striplines required for on-chip spin resonant excitation and field modulation. Electron and hole polarons are injected from opposite sides into the diode structure and recombine spin dependently in the organic semiconductor. ( b , c ) The magnetic field response of a DC current (no modulation) in a bipolar MEH-PPV diode as a function of magnetic field as RF radiation (200 MHz in ( b ); 50 MHz in ( c ) is applied. Reductions in the current are seen when MR conditions are satisfied. These are more pronounced when the applied field B 0 >Δ B Hyp where MR-induced spin mixing dominates. ( d , e ) Schematic illustration of the origin of resistance changes owing to spin mixing induced by the local hyperfine fields (Δ B Hyp ) and owing to MR excitation. All measurements were performed at room temperature. Full size image Resonant current change mechanism First, we scrutinized the assumption that EDMR signals are independent of spin polarization over large magnetic field ranges, a crucial prerequisite for the feasibility of the MRM. For polaron-pair (PP) recombination, spin-dependent rates are based on the spin permutation symmetry of charge carrier pairs, not on spin polarization [19] , [20] , and therefore only a weak B 0 dependence of the signal current is expected. While this model has been scrutinized extensively in recent years with EDMR and ODMR spectroscopy [16] , [21] , [22] , these studies were all performed at X-Band ( B 0 ≈340 mT) [23] or frequencies in the same order of magnitude [24] . Figure 1b,c shows measurements of a direct current flowing through a diode structure as a function of B 0 while a radio frequency (RF) field with constant frequency and amplitude is applied. Figure 1b displays the relative current change Δ I/I in the presence of RF radiation ( ν =200 MHz) as a function of the magnetic field for 1.3 mT< B 0 <10 mT. Throughout the measured range, the plot shows a monotonic increase of the sample current, a behaviour that is due to the strong magnetoresistance. In addition to the monotonic magnetic dependence of the current, the plot displays a current reduction around B 0 ≈7.14 mT, corresponding to the MR condition of g ≈2.0026(4) with a (Δ I/I ≈10 −3 ) decrease of the device current, similar in magnitude to previous X-Band EDMR measurements [16] , [23] . This current change is due to a change of the charge carrier ensembles' spin dynamics from a steady state to a spin-resonantly excited state. When spins of charge carriers are manipulated, the ratio of singlet to triplet pairs changes, and as a result, recombination and dissociation rates, and thus, the current changes, too [16] . We have confirmed this behaviour at a large number of B 0 values between 2 mT and 340 mT, summarized in Fig. 2 . We observed a strong reduction of this differential signal below B 0 ≈2 mT with a detection limit (for a DC measurement with bandwidth ≈10 kHz) at B 0 ≈1 mT. Figure 1c shows the repetition of the measurement illustrated in Fig. 1b for an RF field of ν =50 MHz. Again, a MR-induced change of the current is visible at g ≈2.002 ( B 0 ≈1.79 mT), but with diminished amplitude. We attribute this lower B 0 measurement limit to reduced MR-induced spin-mixing rate changes: as long as the external magnetic field exceeds the local hyperfine field of the π-conjugated polymer ( B 0 > B Hyp ), spin mixing is drastically suppressed and longitudinal spin relaxation rates T 1 are long [25] , [26] . The applied MR can then increase spin mixing artificially (as depicted schematically in Fig. 1d ) [9] , and, therefore, substantially modify the current. In contrast, when B 0 < B Hyp , spin mixing is fast irrespective of MR. Thus, MR changes spin mixing and the spin-dependent current, only marginally, and as a consequence the EDMR signal disappears (as depicted schematically in Fig. 1e ). 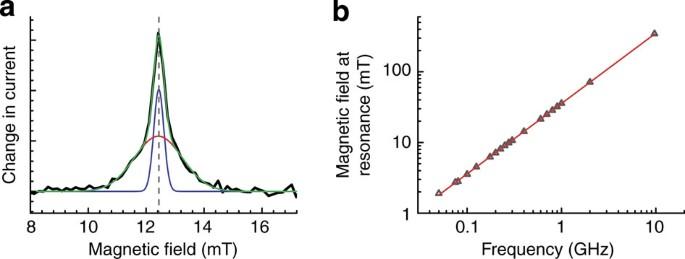Figure 2: Calibration of the MRM. (a) Resonance spectrum for 350 MHz radiation, measured using pulsed resonant excitation. Note that the current change after the excitation pulse was detectable for 1 ms undergoing a quenching/enhancement transient that is known for spin-dependent pair processes35. The data presented here were measured 20 μs after the pulse excitation to maximize signal to noise. The spin resonance used for the MRM device is the narrow (blue) component of the spectrum. The red component represents the wide peak, and the green curve is the fit consisting of the sum of red and blue curves. (b) Plot of the peak magnetic field where maximal MR-induced current change is measured as a function of the applied excitation frequency, following a linear relationship (note that the error of the data points is below the size of the symbols). A linear fit of the above data yields a gyromagnetic ratioγ=28.03(4) GHz T−1and a correspondingg-factorg=2.0026(4). Thus, the electrically detectable electron gyromagnetic ratio can be used as an absolute magnetic field standard. Figure 2: Calibration of the MRM. ( a ) Resonance spectrum for 350 MHz radiation, measured using pulsed resonant excitation. Note that the current change after the excitation pulse was detectable for 1 ms undergoing a quenching/enhancement transient that is known for spin-dependent pair processes [35] . The data presented here were measured 20 μs after the pulse excitation to maximize signal to noise. The spin resonance used for the MRM device is the narrow (blue) component of the spectrum. The red component represents the wide peak, and the green curve is the fit consisting of the sum of red and blue curves. ( b ) Plot of the peak magnetic field where maximal MR-induced current change is measured as a function of the applied excitation frequency, following a linear relationship (note that the error of the data points is below the size of the symbols). A linear fit of the above data yields a gyromagnetic ratio γ =28.03(4) GHz T −1 and a corresponding g -factor g =2.0026(4). Thus, the electrically detectable electron gyromagnetic ratio can be used as an absolute magnetic field standard. Full size image The disappearance of the MR signal when B 0 ≈ B Hyp provides confirmation that the PP (electron-hole) mechanism illustrated in Fig. 1d,e is responsible for both the EDMR signal as well as for the DC magnetoresistance. This assignment has previously been a subject of debate [9] , [23] , [26] , [27] , [28] . It is crucial to note that for MR-based magnetometry, this effect does not set a lower limit on magnetic field measurements: when B 0 < B Hyp , a magnetic field B det = B 0 + B off > B Hyp can be determined by application of a well-defined DC magnetic offset field B off via a direct current in the modulation stripline. B 0 is then obtained from B det − B off . Precision and stability of field sensing Most important for the absolute determination of the magnetic field experienced by our MRM device is the measurement standard, which in this case is the gyromagnetic ratio γ (or Landé g -factor) of the polaron spin. We use the set of EDMR measurements conducted on our thin-film samples over a large magnetic field range in order to accurately determine γ and to confirm the independence of γ from the magnetic field itself. We note that ODMR through luminescence detection could be used for this in an identical way [21] ; however, as on-chip light detection within an organic semiconductor device is technically much more demanding than current detection, we focus solely on EDMR measurements. Experimentally, we used B 0 -dependence measurements for single-pulse transient experiments. One fitted spectrum for ν =350 MHz is shown as an example in Fig. 2a . As expected for the EDMR spectrum of the PP process, the signal shows two Gaussian peaks corresponding to the two charge carrier species [16] , [21] . In order to maximize the accuracy of the B 0 measurement, we chose the narrow Gaussian peak for the MRM, which is attributed to one charge carrier species (electron or hole). Figure 2b displays a plot of the magnetic field values for which the maximal current change was observed as a function of the applied RF field. The data are fit by a linear function revealing a value of γ =28.03(4) GHz T −1 . The slight difference between this value and the free-electron gyromagnetic ratio (28.025 GHz T −1 ) arises owing to the weak but non-negligible spin–orbit coupling of the charge carrier spin states [22] , [29] . Figure 2b demonstrates the reproducibility of this value over nearly three orders of magnitude in MR frequency (40 MHz–9.7 GHz). The limitation of our experiment to <≈340 mT (≈9.7 GHz) is of purely technical nature. To determine the operational range of our sensor, we have explored the stability of the gyromagnetic ratio in our devices as a function of temperature and intentional device degradation. This determination was accomplished by reproducing γ at a collection of temperatures ranging from 5 K to room temperature, and repeating the experiment after deliberate device degradation. The results of these experiments are summarized in Fig. 3a, which shows the gyromagnetic ratios obtained under the different conditions. Note that the error bars displayed for each of the data points represent the standard deviation estimated from the fit of the EDMR spectra belonging to the individual measurements. The true errors are expected to be much lower than these fit estimates as the variation of the data throughout the measurement range is much smaller. To test this hypothesis, we compared the temperature average value ( γ =28.03 GHz T −1 represented by the red line) with its standard deviation obtained from the entire set of measurements ( σγ =0.01 represented by the grey bar about the red line). This comparison shows that the real error of the individual measurements is about 10 MHzT −1 and that within this error, the magnetic field measurement is independent of temperature over almost two orders of magnitude; and that we have a confirmation of γ when compared with the fit in Fig. 2 . 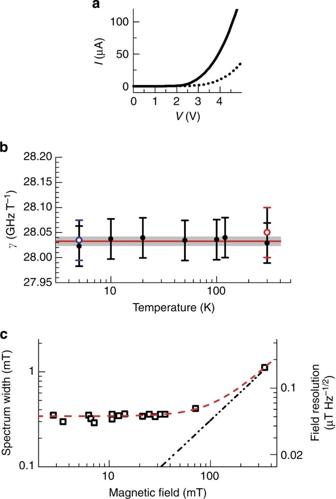Figure 3: Robustness and sensitivity limits of the magnetometer device. (a) The current–voltage characteristics of a device at 5 K before (solid line) and after (dashed line) intentional significant degradation in air. (b) The gyromagnetic ratio,γ, measured as a function of temperature and degradation. The closed points derive from pristine devices and the open circles (with coloured error bars) from two of these devices after degradation. The error bars are upper estimates obtained from the fits of the individual spectra. The grey bar represents the s.d. obtained from all data points. The red solid line gives the temperature average of all data. Within this range, neither the change in temperature nor degradation of the materials impact the reproducibility of the gyromagnetic ratio. (c) Plot of the MR peak width (left axis) as well as the resulting field resolution (right axis) as a function of the externally applied magnetic field. The data belong to both the left and right axis. At low magnetic fields, the hyperfine interaction dominates the resonance widths while spin-orbit contributions (which causeg-factor inhomogeneities) dominate at high magnetic fields leading to spectral broadening. The dashed red line represents a fit of the data with both hyperfine field strength and spin-orbit (g-factor) distribution. The dashed black line shows the spin-orbit-induced broadening obtained from the fit of the data. Figure 3: Robustness and sensitivity limits of the magnetometer device. ( a ) The current–voltage characteristics of a device at 5 K before (solid line) and after (dashed line) intentional significant degradation in air. ( b ) The gyromagnetic ratio, γ , measured as a function of temperature and degradation. The closed points derive from pristine devices and the open circles (with coloured error bars) from two of these devices after degradation. The error bars are upper estimates obtained from the fits of the individual spectra. The grey bar represents the s.d. obtained from all data points. The red solid line gives the temperature average of all data. Within this range, neither the change in temperature nor degradation of the materials impact the reproducibility of the gyromagnetic ratio. ( c ) Plot of the MR peak width (left axis) as well as the resulting field resolution (right axis) as a function of the externally applied magnetic field. The data belong to both the left and right axis. At low magnetic fields, the hyperfine interaction dominates the resonance widths while spin-orbit contributions (which cause g -factor inhomogeneities) dominate at high magnetic fields leading to spectral broadening. The dashed red line represents a fit of the data with both hyperfine field strength and spin-orbit ( g -factor) distribution. The dashed black line shows the spin-orbit-induced broadening obtained from the fit of the data. Full size image Even with encapsulation, devices made with organic semiconductors can degrade over time, leading to fluctuations in device conductivity. We have simulated the effect of this degradation by exposing our diodes to ambient atmosphere for 24 h [30] , without using any protective measures, to investigate the impact of degradation on the MR approach described above. The comparison of the current voltage characteristics of the degraded and the pristine sample is shown in Fig. 3a . The curves exhibit a strong reduction in device conductivity upon deterioration, which impacts on DC magnetoresistance. In contrast to this significant device modification, the resonant current change occurs under the same gyromagnetic ratio after degradation. Within the error determined from the pristine sample, the MRM is entirely insensitive to degradation. We repeated the measurements of γ on different thin-film samples made with a variety of contact materials (with a range of work functions) as well as with different spin-casting parameters. The results of these measurements indicate that while the gyromagnetic ratio of the two resonance lines can vary for different contact and active materials, the temperature independence and degradation independence for any given sample is reproduced for the narrow resonance line that is used for magnetometry. We also note that we did not observe any line shape or g -factor dependence on applied bias, which further corroborates the robustness of our magnetic field standard. We discuss next the sensitivity limitations of the organic MRM. Using field-modulated lock-in detection, the lower limit of the distinguishable field strength, or the minimum resolved external field [8] δB min , depends on the spectral line width, the electrical shot noise [31] and the modulation amplitude of the driving field in the following form: where and B m is the amplitude of modulation. The second derivative of the magnetic field-dependent current, as given in the denominator of this term, represents the 'sharpness' of the resonance used, that is, the slope (the first derivative) of the lock-in-detected spectrum at the zero-crossing point. As this quantity is the second derivative of a Gaussian for the hyperfine-field-broadened resonance [16] , it is proportional to the line width. The widths of the EDMR spectra, and thus the device sensitivity, are not always independent of external magnetic field. EDMR lines can be broadened inhomogeneously (randomly, following a Gaussian) owing to a distribution of spin–orbit interactions as well as hyperfine fields. Intersite variations in spin–orbit interaction lead to a distribution of the g -factor, and therefore a resonance line width proportional to the applied B 0 field. In contrast, inhomogeneous broadening due to random hyperfine fields is independent of any external magnetic field as long as the nuclear spin ensemble remains unpolarized by the external field (at room temperature, significant thermal hydrogen nuclear polarization cannot be achieved with static magnetic fields <100 T). Thus, for the polaron resonance line used here, at low external magnetic fields we expect the line widths to be limited by random hyperfine fields, and therefore to be constant. As spin–orbit-induced line broadening exceeds the hyperfine fields, the linewidth should become proportional to the external magnetic field. Figure 3c , left ordinate (red line), displays the measured line width of the PP resonance as a function of B 0 . When hyperfine fields and spin–orbit effects convolute, we expect the Gaussian line width Δ B to be the geometric sum of the hyperfine field distribution width B Hyp and the spin–orbit-induced width of the gyromagnetic ratio α multiplied by the applied external magnetic field B 0 . The fit of the data in Fig. 3c with this relation reveals B Hyp ∼ 0.35 mT (note that only the narrow polaron line was used here) while α ≈2.9×10 −3 is given by the line width obtained from a linear fit of the data at high fields where the spin–orbit term dominates. This value is in excellent agreement with a previous estimate of the spin–orbit-induced variations in g -factor based on X-band MR [28] . Given these parameters, we can now estimate the resolution limit for the MEH-PPV devices used in this study. For a modulation amplitude B m =Δ B =0.35 mT, a device current of I 0 =100 μA and a MR-induced current change of I A =100 nA, we obtain a resolution of δ B min ∼ 50 nT Hz −1/2 with unity signal to noise within the hyperfine-limited magnetic field range (<100 mT). The resolution for larger B 0 is given in Fig. 3c , right ordinate (black line). An integrated MR-based organic magnetometer In order to measure an externally applied magnetic field B 0 , changes to a current flowing through the diode structure are monitored by a lock-in amplifier whose reference frequency is provided by a low-frequency alternating current that is applied to a thin-film stripline 'coil' that is positioned underneath the diode. This lock-in-detected current change is then measured as a function of the RF field applied to a second thin-film stripline positioned underneath the first stripline with perpendicular orientation (the B 1 field). Once a frequency ν is identified at which the MR-induced diode current change is maximized, finding B 0 = ν / γ is simple, with γ being the gyromagnetic ratio of the charge carrier species that is in resonance. The results described above confirm that the spin-dependent PP mechanism in MEH-PPV exhibits the resonance and stability properties that are needed for an organic semiconductor MRM. We now demonstrate that all required components—the organic diode, magnetic field modulation and a method for generating a resonant microwave frequency—can be integrated into a monolithic device, as sketched in Fig. 1a . A diode, used to measure MR current changes, sits near two thin perpendicular strips of conducting materials, which are electrically isolated from each other. One of the strips, the resonance stripline, is coupled to a high-frequency source (low megahertz to gigahertz range) that is used to generate the oscillating magnetic field required for spin resonance. A current is applied to the other strip to generate a magnetic field, either oscillating (to enable lock-in detection) or static (for offsetting the resonance field, for example, to shield out B Hyp ), or both. We have used this device to perform real magnetometry experiments. To determine the magnetic field B 0 , a sweep of the frequency is carried out until the MR condition is found. As it is difficult to design a stripline with constant transmission properties over a very wide range of frequencies, we use a magnetic field modulation lock-in scheme to filter the effects of the unwanted current changes that result from the coupling between the resonance strip and the device. During a measurement, the MR excitation frequency is stepped on one line while a low-frequency (kHz) magnetic field modulation is applied to the other. Lock-in detection is then used to monitor changes in the device current. 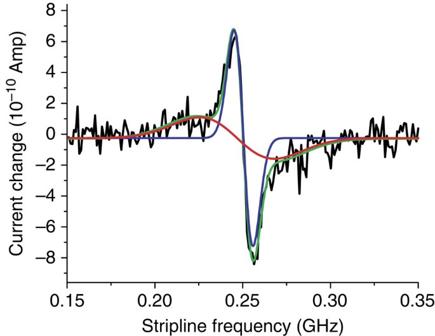Figure 4: An integrated absolute magnetic field sensor. The magnetic field-modulated current change in an integrated device as sketched inFig. 1aas a function of stripline frequency in a static magnetic field of 8.93 mT. A small modulation field of 0.05 mT is applied to the static field at a frequency of 6 kHz via the second stripline (labelledBmodinFig. 1a) to enable lock-in detection. The data show the presence of two Gaussian resonances (red and blue curves), with the narrow resonance (blue fit) being significantly more pronounced in the lock-in-detected derivative spectrum. Note that the presence of the broader of the two resonance lines (red) does not compromise the measurement as both resonances exhibit identical gyromagnetic ratios. The green curve represents the fit of the data using the sum of the two Gaussians. Figure 4 shows the B 0 -modulated device current change as the RF field is swept while the external magnetic field is held at a constant, arbitrary value. As we now employ lock-in detection, the derivative spectrum of the resonance line is seen. The zero crossing of the measured function is observed at 250.5(1) MHz, corresponding to a B 0 =8.93(2) mT. From this data, we determined a sensitivity spectral density of 6 μT Hz −1/2 . This agrees with the relation for δB min given above, with B m ∼ 0.05 mT and a bandwidth of Δ f ∼ 10 Hz. Figure 4: An integrated absolute magnetic field sensor. The magnetic field-modulated current change in an integrated device as sketched in Fig. 1a as a function of stripline frequency in a static magnetic field of 8.93 mT. A small modulation field of 0.05 mT is applied to the static field at a frequency of 6 kHz via the second stripline (labelled B mod in Fig. 1a ) to enable lock-in detection. The data show the presence of two Gaussian resonances (red and blue curves), with the narrow resonance (blue fit) being significantly more pronounced in the lock-in-detected derivative spectrum. Note that the presence of the broader of the two resonance lines (red) does not compromise the measurement as both resonances exhibit identical gyromagnetic ratios. The green curve represents the fit of the data using the sum of the two Gaussians. Full size image The position of the resonance, and thus the measured magnitude of the field, is independent of the orientation of the sensor. However, the amplitude of the resonant change in current for unknown fields oriented parallel to B 1 will be vanishingly small. This does not pose a limitation on the device, as it is possible to use either one of the perpendicular strips for driving spin resonance. Along with the magnitude, the direction of the measured magnetic field can then be determined by adding small offset fields and repeating the measurement, allowing the use of simple geometric analysis to determine the orientation of the magnetic field. We have demonstrated a calibration and offset-free, temperature- and degradation-independent, MR-based organic thin-film magnetometer. We illustrated the feasibility of this sensor for magnetic fields B 0 in a range 1 mT< B 0 <340 mT. These are not fundamental limitations, but more technical in nature. The upper limit was set by our microwave frequency equipment, while the lower limit can be overcome by a DC offset field added to the B 0 modulation. We have integrated the sensor into a monolithic device capable of high precision sensing. We anticipate that, owing to the all-thin-film design of the device, a large number of sensors could be accommodated on a single (perhaps flexible) substrate for imaging spatially varying magnetic fields [32] , with a spatial resolution of <100 nm [33] . A comparison of this organic MRM concept with existing magnetometer devices (discussed in detail elsewhere [34] ) shows that this implementation may fill the gap for intermediate-field precision magnetometry on small length scales. The organic MRM is less sensitive than SQUIDs but more sensitive than Hall sensors. In contrast to SQUIDs, which only work at cryogenic temperatures, and Hall sensors, whose calibration is very temperature-dependent, the organic MRM operates—calibration free—over large temperature ranges. Compared with conventional NMR-based MRMs, which are bulky and have diminished sensitivity in the lower magnetic field range, the organic MRM can be very small and its sensitivity is independent of magnetic field over a wide range. As NMR resonances are narrower than the polaron resonance used for the organic MRM, NMR-based MRMs will provide higher sensitivity at high magnetic fields. Similarly, for very small magnetic fields, SQUIDs will continue to be the most sensitive magnetic field detectors. We note that MRMs using nitrogen-vacancy centres in diamond have a number of the advantages discussed here (such as good temperature stability and high spatial resolution), but unlike the OLED-based magnetometer, they cannot be accessed electrically. The most significant challenge for the organic thin-film MRM could be the time required to find the MR reference frequency. As for conventional NMR-based MRMs, this can require time-consuming frequency sweeps. However, for the proposed device design, this drawback could potentially be overcome by a combination of the MRM operation mode of the device with the magnetoresistive behaviour of the polymer layer. This approach would enable magnetic fields to be measured at high bandwidth using the magnetoresistance effect, while the MRM mode is used periodically for recalibration. As recalibration of the magnetoresistive sensor would be needed only occasionally to compensate for degradation and strong temperature changes, this organic hybrid magnetometer would, in essence, combine the advantages of both sensor approaches: the speed of a magnetoresistive measurement with the temperature and degradation-independent accuracy of an MRM. Significantly increased sensitivity could also be obtained by exploiting the long spin phase coherence found in these materials, to perform quantum-enhanced field sensing [14] , [35] , although this would require more complex pulsed spin resonance excitation [35] . Device fabrication The EDMR device is a diode [36] stack consisting of the following materials: an indium tin oxide layer of ∼ 200 nm, a hole injection layer of poly(3,4-ethylenedioxythiophene) ( ∼ 50 nm thick) that was applied using a spin coater at ∼ 3,000 r.p.m., a thin layer ∼ 200 nm of MEH-PPV with density ∼ 7.5 g l −1 in chlorobenzene that was also applied via spin coating at ∼ 1600 r.p.m. in a nitrogen glove box and a ∼ 25-nm-thick calcium contact to ensure good electron injection, followed by an Al layer ( ∼ 50 nm thick). Devices were fabricated on Corning glass substrates. The temperature-dependent γ data were taken with devices with either Sr or Ca electrical top contacts in order to verify the contact material independence of the observed spectra. The Al, Ca and Sr contacts were thermally evaporated in a nitrogen glove box at a pressure of ∼ 10 −6 mbar. Experimental setup For the measurements in Fig. 1b,c , the device was operated in forward bias with a SRS SIM928 isolated voltage source, and placed inside a small coil. The coil was connected to a tunable frequency source for the application of a fixed frequency. The device output current was then connected to an SRS SR570 low-noise current amplifier set to operate as a low-pass filter (10 Hz cutoff). The output then connected to a 16-bit fast digitizer card for acquisition. For the single pulse experiments included in Fig. 2 , a single stripline resonator design was used while the diode was operated in forward bias mode. The output current was then connected to a SRS SR570 low-noise current amplifier in high-bandwidth mode with an offset current close to I 0 . This output was then connected to an 8-bit transient recorder. For the data in Fig. 4 , the device was operated in forward bias while situated close to two electrically separated stripline resonators (as described in Fig. 1a ) for the application of the driving and modulation fields, respectively. A reference frequency of ∼ 6 kHz was fed to the modulation stripline by a SRS DS345 function generator at ∼ 5V pp thus providing ∼ 0.02 mT of modulation field amplitude. The in-phase output was then connected to a 16-bit fast digitizer card for data acquisition. The stripline resonators consisted of copper strips on either side of an epoxy substrate. Simple mechanical contact of the OLED device to the stripline circuit board was sufficient to induce a resonance. Sensitivity analysis The sensitivity (also called resolution) δB min of an individual magnetic field measurement corresponds to the error (the s.d.) of a single measurement. Its unit is equal to the unit of the observed quantity, the magnetic field. If conducting a measurement with sensitivity δB min takes a time τ , then the sensitivity of the setup can be improved to a sensitivity simply by conducting n measurements in a time nτ followed by averaging of the n measured values. The sensitivity of a magnetometer is therefore dependent on the measurement time and it is more meaningful to describe the device in terms of its sensitivity spectral density (which, rather confusingly, is often also referred to as 'sensitivity' in the literature). The sensitivity spectral density is a magnetic field times the square root of time, its unit is [T√s]=[T/√Hz]. The sensitivity δB min of the MRM magnetometer discussed here can be affected by the electrical shot noise, the amplitude of the applied modulation field B m and the width of the resonance line Δ B through the following relation: where is the shot noise. is the second derivative of the magnetic field dependence of the device current I ( B 0 ), which for the case of MEH-PPV is a Gaussian function with I a being the spin-dependent on-resonance signal current through the device. Δ f is the bandwidth of the measured signal and is defined by the low-pass filter of the lock-in detector. At the centre of the Gaussian distribution ( B 0 =B res ), Thus, the sensitivity spectral density is where we have assumed that the modulation amplitude B m is set equal to the line width Δ B . For the resolution estimation in the given devices, we used experimental values of I a =100 nA, I 0 =100 μA and Δ B =0.35 mT as obtained from the fits in Fig. 3c . How to cite this article: Baker, W.J. et al . Robust absolute magnetometry with organic thin-film devices. Nat. Commun. 3:898 doi: 10.1038/ncomms1895 (2012).